Electrical control of neutral and charged excitons in a monolayer semiconductor Monolayer group-VI transition metal dichalcogenides have recently emerged as semiconducting alternatives to graphene in which the true two-dimensionality is expected to illuminate new semiconducting physics. Here we investigate excitons and trions (their singly charged counterparts), which have thus far been challenging to generate and control in the ultimate two-dimensional limit. Utilizing high-quality monolayer molybdenum diselenide, we report the unambiguous observation and electrostatic tunability of charging effects in positively charged (X + ), neutral (X o ) and negatively charged (X − ) excitons in field-effect transistors via photoluminescence. The trion charging energy is large (30 meV), enhanced by strong confinement and heavy effective masses, whereas the linewidth is narrow (5 meV) at temperatures <55 K. This is greater spectral contrast than in any known quasi-two-dimensional system. We also find the charging energies for X + and X − to be nearly identical implying the same effective mass for electrons and holes. Above bandgap photo-excitation creates electrons and holes in the conduction and valence bands, respectively. If the screening is weak enough, the attractive Coulomb interaction between one electron and one hole creates a bound quasi-particle known as a neutral exciton (X o ), which has an energy structure similar to a neutral hydrogen atom. Excitons can further become charged by binding an additional electron (X − ) or hole (X + ) to form charged three-body excitons analogous to H − or H 2 + respectively [1] , [2] , [3] . These exciton species are elementary quasi-particles describing the electronic response to optical excitation in solids and are integral to many optoelectronic applications from solar cells and light-emitting diodes [4] to optical interconnects [5] and quantum logical devices [6] , [7] . The main arena for the exploration of excitonic physics has been three-dimensional semiconductors and their heterostructures that form quasi-2D quantum wells where the carrier wavefunction typically occupies a few tens to thousands of atomic layers. Observation and control of excitons in truly 2D systems has been a long pursued goal, largely motivated by the enhancement in exciton- and trion-binding energies in the strict 2D limit [8] . In addition, unlike semiconductor heterostructures, the close proximity of external stimuli to the exciton wavefunction can offer unprecedented tunability and diversifies the applications possible in devices made with 2D semiconductors. Here we report the experimental observation and control of the fascinating excitonic physics in a 2D semiconductor by utilizing high-quality monolayer molybdenum diselenide (MoSe 2 ). MoSe 2 belongs to the group-VI transition metal dichalcogenides, which form in layers weakly bound to each other by Van der Waals forces. The monolayers have received much attention recently as they make up a new class of 2D semiconductors with a direct bandgap in the visible frequency range and are predicted to exhibit coupled spin-valley physics [9] . Recent progresses focus on MoS 2 , including the demonstration of having a direct bandgap [10] , [11] , high mobility electronics [12] , optical generation of valley polarization [13] , [14] , [15] and electrical control of Berry phase properties [16] . Using a back-gated field-effect transistor (FET) device, we demonstrate the reversible electrostatic tunability of the exciton charging effects from positive (X + ) to neutral (X o ) and to negative (X − ). We observe a large trion-binding energy of 30 meV with a narrow emission linewidth of 5 meV. These narrow, well-separated features have temperature dependence of typical 2D excitons and exist at high temperature suggesting remarkable stability. Interestingly, the binding energies of X + and X − are similar implying that low-energy electrons and holes in MoSe 2 have the same effective mass. Our work demonstrates that monolayer MoSe 2 is a true 2D semiconductor opening the door for the investigation of phenomena such as exciton condensation [17] , [18] , [19] and the Fermi-edge singularity [20] , [21] , as well as for a new generation of optoelectronic devices such as light-emitting diodes and excitonic circuits [5] . Crystal structure and spectral features of monolayer MoSe 2 In monolayer MoSe 2 , Mo and Se atoms form a 2D hexagonal lattice with trigonal prismatic coordination ( Fig. 1a ). First-principles calculations show that it has a direct bandgap at the corners (K points) of the first Brillouin zone ( Fig. 1b ). The curvature of the bands suggests comparable effective mass for low-energy electrons and holes at K points ( Fig. 1c ) [9] . These band-edge electrons and holes near K points are predominantly from the d -orbitals of Mo atoms. Their wavefunctions are calculated to be strongly confined in the Mo layer within a length scale of ~0.2 nm in the out-of-plane direction. Monolayer MoSe 2 is thus an ideal nanomaterial for exploring excitonic physics in the ultimate 2D limit. 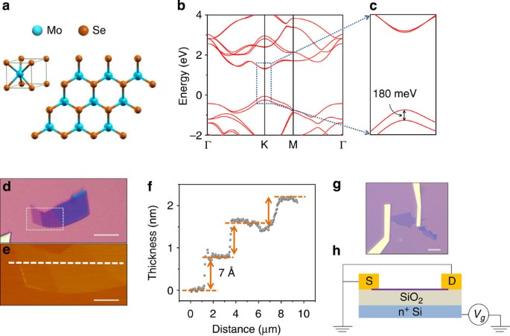Figure 1: MoSe2characteristics and devices. (a) Coordination structure and top view of monolayer MoSe2. (b) Density function theory calculated band structure. (c) Band structure at K point shows 180 meV valence band splitting due to spin–orbit coupling. (d) Optical micrograph of exfoliated MoSe2flake on 300 nm SiO2. Scale bar, 5 μm. (e) atomic force microscope (AFM) image of area highlighted in (d). Scale bar, 1 μm. (f) AFM line scan along dashed line ine. (g) Optical micrograph of MoSe2device. Scale bar, 5 μm. (h) Schematic of back-gated MoSe2device. Figure 1: MoSe 2 characteristics and devices. ( a ) Coordination structure and top view of monolayer MoSe 2 . ( b ) Density function theory calculated band structure. ( c ) Band structure at K point shows 180 meV valence band splitting due to spin–orbit coupling. ( d ) Optical micrograph of exfoliated MoSe 2 flake on 300 nm SiO 2 . Scale bar, 5 μm. ( e ) atomic force microscope (AFM) image of area highlighted in ( d ). Scale bar, 1 μm. ( f ) AFM line scan along dashed line in e . ( g ) Optical micrograph of MoSe 2 device. Scale bar, 5 μm. ( h ) Schematic of back-gated MoSe 2 device. Full size image We use mechanical exfoliation to obtain monolayer MoSe 2 on 300 nm SiO 2 on n + -doped Si and atomic force microscope to identify the layer thickness [22] . Figure 1d show the optical micrograph and the corresponding atomic force microscope image of a representative sample, in which the monolayer thickness of ~0.7 nm is identified [12] ( Fig. 1f ). Standard electron beam lithography (EBL) is used to fabricate monolayer FETs ( Fig. 1g ). With the contacts simply grounded, the n + Si functions as a back gate providing uniform electrostatic doping in the MoSe 2 ( Fig. 1h ). The excitonic features of MoSe 2 are investigated by differential reflectance and micro photoluminescence (PL) measurements (Methods). 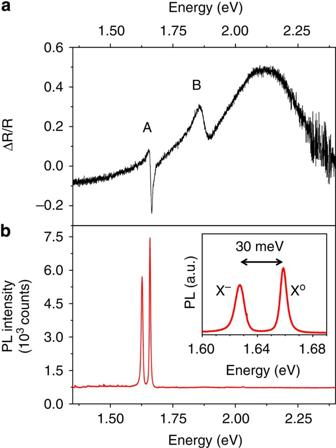Figure 2: Differential reflectance and PL spectra of monolayer MoSe2at 20 K. (a) Differential reflectance shows A and B excitons. (b) PL excited by 2.33 eV laser shows neutral exciton (Xo) and the lower-energy charged exciton (X−). PL from the B exciton has not been observed. Inset, PL of the exciton peaks. The X−shows a binding energy of about 30 meV. Figure 2 shows the results from an unpatterned MoSe 2 sample, S1. At 20 K, we observe two main features associated with the A and B excitons in the differential reflection spectrum [10] , [11] , [14] , [23] , [24] , [25] ( Fig. 2a ). The presence of A and B excitons has been attributed to spin–orbit coupling-induced valence band splitting in bulk [24] . The observed energy difference of ~200 meV agrees well with the calculated splitting (180 meV) in monolayers ( Fig. 1c ). Figure 2: Differential reflectance and PL spectra of monolayer MoSe 2 at 20 K. ( a ) Differential reflectance shows A and B excitons. ( b ) PL excited by 2.33 eV laser shows neutral exciton (X o ) and the lower-energy charged exciton (X − ). PL from the B exciton has not been observed. Inset, PL of the exciton peaks. The X − shows a binding energy of about 30 meV. Full size image With the same sample and temperature under 2.33 eV laser excitation, the PL spectrum does not show a measurable feature that can be attributed to the B exciton, likely because it is not the lowest energy transition. Instead, we observe two pronounced peaks at 1.659 and 1.627 eV in the vicinity of the A exciton ( Fig. 2b ). Note that the PL spectrum lacks the broad low-energy peak observed in MoS 2 , which has been attributed to defect-related, trapped exciton states [10] , [11] , [14] , [25] . The striking spectral features demonstrate the high quality of our MoSe 2 samples (Methods) and provide strong evidence for monolayer MoSe 2 being a direct bandgap semiconductor ( Supplementary Fig. S1 ) where the two distinct transitions are excitons. The higher-energy emission at 1.659 eV is the neutral exciton, X o , and the lower-energy peak is a trion [3] . In unpatterned samples, we assume the trion to be X − because all measured devices show n-doped characteristics ( Supplementary Fig. S2 ). All measured unpatterned samples show a binding energy, which is the energy difference between trion and X o , of ~30 meV ( Fig. 2b , inset). This is more than twice the typical numbers reported in GaAs quantum wells [3] , [26] , [27] and similar to a recent mention in MoS 2 [14] . Gate dependence of MoSe 2 PL To confirm the above assignment and control the exciton charging effects, we performed gate-dependent PL measurements using monolayer MoSe 2 FETs. Here the excitation laser is at 1.73 eV for better resonance with the luminescent states. 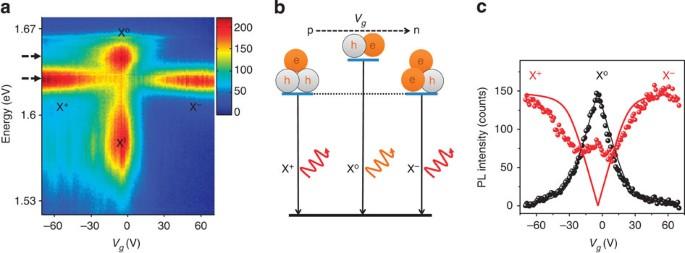Figure 3: Electrostatic control of exciton charge. (a) MoSe2PL (colour scale in counts) is plotted as a function of back-gate voltage. Near zero doping, we observe mostly neutral and impurity-trapped excitons. With large electron (hole) doping, negatively (positively) charged excitons dominate the spectrum. (b) Illustration of the gate-dependent trion and exciton quasi-particles and transitions. (c) Trion and exciton peak intensity versus gate voltage at dashed arrows in (a). Solid lines are fits based on the mass action model. Figure 3a shows a colour map of the PL spectrum of device D1 at 30 K as a function of back-gate voltage, V g , in which we clearly observe four spectral features whose intensities strongly depend on V g . Near zero V g , the spectrum shows a broad low-energy feature around 1.57 eV and a narrow high-energy peak at 1.647 eV. With large V g of either sign, these peaks disappear and a single-emission peak dominates the spectrum. Both peaks (at negative or positive V g ) have similar energies and intensities with the latter increasing with the magnitude of V g . Figure 3: Electrostatic control of exciton charge. ( a ) MoSe 2 PL (colour scale in counts) is plotted as a function of back-gate voltage. Near zero doping, we observe mostly neutral and impurity-trapped excitons. With large electron (hole) doping, negatively (positively) charged excitons dominate the spectrum. ( b ) Illustration of the gate-dependent trion and exciton quasi-particles and transitions. ( c ) Trion and exciton peak intensity versus gate voltage at dashed arrows in ( a ). Solid lines are fits based on the mass action model. Full size image This observed gate dependence confirms the assignment of states as labelled in Fig. 3a . Because the broad low-energy peak does not show up in unpatterned samples before FET fabrication, we attribute it to exciton states trapped to impurities (X I ) [10] , [11] , [14] , [25] , which are likely introduced during EBL processing and are not the focus of this paper. The sharp peak at 1.647 eV is the X o , slightly red-shifted compared with unpatterned samples. From the gate dependence, we identify the peaks near 1.627 eV as the X − and X + trions when V g is largely positive and negative, respectively. Remarkably, these two distinct quasi-particles (X + and X − ) exhibit a nearly identical binding energy. The difference is within 1.5 meV over the whole applied V g range. Because the binding energy of a trion is dependent on its effective mass, this observation implies that the electron and hole have approximately the same effective mass. The gate-dependent measurements unambiguously demonstrate the electrical control of exciton species in a truly 2D semiconductor, as illustrated in Fig. 3b . The conversion from X o to trion can be represented as e(h)+X o →X − (X + ), where e and h represent an electron or a hole, respectively. By setting V g to be negative, the sample is p-doped, favouring excitons to form lower-energy-bound complexes with free holes. As V g decreases, more holes are injected into the sample, and all X o turn into X + to form a positively charged hole-trion gas. With positive V g , a similar situation occurs with free electrons to form an electron-trion gas. In the following, we show that a standard mass action model can be used to describe the conversion dynamics. Figure 3c shows the extracted X o (black) and trion (red) peak intensity as a function of V g where we have adjusted the negative V g data due to background signal. The plot shows that the maximum X o intensity is about equal to the saturated trion PL when X o vanishes. This observation indicates conservation of the total number of X o and trion in the applied voltage range and similar radiative decay rates for both quasi-particles. Thus, the PL intensity represents the amount of the corresponding exciton species. Because the dynamic equilibrium of free electrons, holes and excitons are governed by the rate equation and law of mass action [27] , we calculate the gate-dependent X o and trion abundance ( Supplementary Fig. S3 ), shown by the solid lines in Fig. 3c , which agrees with the data. In the simulation, we first fit the X o curve to obtain our two free parameters: the maximum background electron concentration when the trion intensity saturates and the photo-excited electron concentration n p =1.5 × 10 10 cm −2 . We then fit the trion gate dependence with these parameters held fixed ( Supplementary Note 1 ). The deviation in the trion experimental data from the calculated curve near zero V g is artificial due to the mutual background from X o and X I . We note that this inferred electron concentration is much smaller than the product of the gate capacitance and V g . This discrepancy can be attributed to the large contact resistance ( Supplementary Fig. S4 ) of the sample, which prevents the carrier concentration from reaching equilibrium on the experimental time scale at 30 K. We expect that future improved contact technologies will eliminate this effect. Temperature dependence of MoSe 2 PL The observed exciton states also show fine features consistent with 2D excitons, such as temperature-dependent line shape, peak energy and relative weight of X o and trion, which further supports the excitonic nature of this monolayer system ( Fig. 4 ). 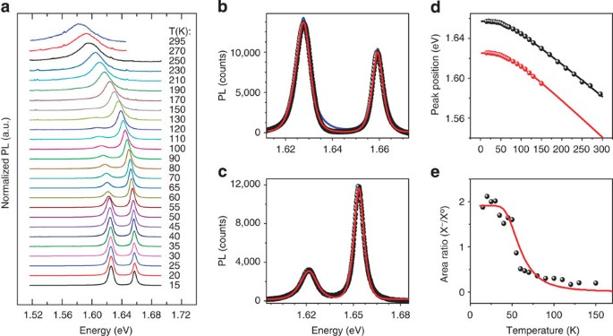Figure 4: Temperature dependence of PL spectrum. (a) Normalized PL of monolayer MoSe2versus temperature. (b) Line shape fitting at 15 K. Black is data. Red and blue curves are fits with and without considering the electron-recoil effect, respectively. (c) Data and fit at 70 K using two symmetric peaks. (d) Neutral exciton (black) and trion (red) peak position versus temperature with fits (solid lines). (e) Integrated area ratio of trion:exciton versus temperature with mass action model fitting (red). Figure 4a shows the evolution of X − and X o (normalized PL) as a function of temperature in an unpatterned sample, S2, under 1.96 eV laser excitation. At low temperatures, we again observe a binding energy of 30 meV. As the temperature rises, we see the X − signal drop significantly at about 55 K, which we attribute to electrons escaping their bound trion state due to thermal fluctuations ( Supplementary Note 1 ). Figure 4: Temperature dependence of PL spectrum. ( a ) Normalized PL of monolayer MoSe 2 versus temperature. ( b ) Line shape fitting at 15 K. Black is data. Red and blue curves are fits with and without considering the electron-recoil effect, respectively. ( c ) Data and fit at 70 K using two symmetric peaks. ( d ) Neutral exciton (black) and trion (red) peak position versus temperature with fits (solid lines). ( e ) Integrated area ratio of trion:exciton versus temperature with mass action model fitting (red). Full size image Figure 4b is the zoom-in plot at 15 K where we observe slightly different line shapes for X − and X o . The X o peak is symmetric showing homogenous thermal broadening effects and is well fit by a hyperbolic secant function that yields a full-width half-maximum of 5 meV [27] , [28] . However, the X − peak shows a slightly asymmetric profile with a long low-energy tail consistent with electron-recoil effects [27] . The recombination of a X − with momentum k will emit a photon and leave a free electron with the same momentum k due to momentum conservation. From energy conservation, the emitted photon has an energy , where is the energy of trions with k =0, and and are the X o and X − effective masses, respectively. The line shape of trion PL will thus be the convolution of a symmetric peak function (hyperbolic secant) and an exponential low-energy tail function ( Supplementary Fig. S5 and Supplementary Note 2 ). When the temperature is >70 K, we find that homogenous broadening dominates over electron recoil and the PL spectrum is fit well by two hyperbolic secant functions ( Fig. 4c ). From the fits, we extract the X − and X o peak position ( Fig. 4d ) and the ratio of the integrated intensity of the X − to the X o ( Fig. 4e ) where we do not present trion data >150 K because it becomes negligible. We find that the peak positions are fit well (solid line in Fig. 4d ) using a standard semiconductor bandgap dependence [29] of , where E g (0) is the ground-state transition energy at 0 K, S is a dimensionless coupling constant and is an average phonon energy. From the fits, we extract for X o (X − ) the E g =1.657 (1.625) eV, S =1.96 (2.24) and 15 meV for both. Applying our mass action model ( Supplementary Fig. S3 and Supplementary Note 1 ) with a trion-binding energy of 30 meV results in a good fit to the X − :X o intensity ratio (solid line in Fig. 4e ). In summary, we have shown that monolayer MoSe 2 is a true 2D excitonic system, which exhibits strong electrostatic tuning of exciton charging via a standard back-gated FET. The observed narrow, well-separated spectral features are within the titanium (Ti)-Sapphire laser spectral range and thus provide remarkable opportunities to selectively probe and control specific excitons using current continuous wave and ultrafast Ti-Sapphire laser technologies. Our results further demonstrate that high-quality monolayer dichalcogenides can serve as a platform for investigating excitonic physics and photonic applications in the truly 2D limit with the potential to outperform quasi-2D systems. The results represent unique prospects for this burgeoning class of 2D materials, in addition to the recent attention received for their valley physics. Our work expands the horizons for using 2D semiconductors for diverse fundamental studies and technical applications. Note: During the review process, we became aware of the independent observation of negatively charged exciton in monolayer MoS 2 (ref. 30 ) and investigation of PL intensity of thin-film MoSe 2 as a function of temperature [31] . Sample growth MoSe 2 single crystals were grown by vapour transport. First, MoSe 2 powder was prepared by heating a stoichiometric mixture of Mo (Alfa, 99.999%) powder and Se (Alfa, 99.999%) pieces sealed in a quartz tube under 1/3 atmosphere of pure argon. The ampoule was slowly heated up to 850 °C and kept at this temperature for 24 h. Then, 3.5 g of MoSe 2 powder was mixed with 0.5 g of iodine and sealed in a quartz tube. The sealed ampoule was loaded into a tube furnace for 10 days, with the hot zone kept at 1,050 °C and the growth zone at 1,000 °C. Plate-like crystals with typical dimensions 6 × 10 × 0.1 mm 3 were obtained at the cold end. Room-temperature X-ray diffraction confirmed that the samples are single phase with 2H structure. Elemental analysis was performed using a Hitachi TM-3000 tabletop electron microscope equipped with a Bruker Quantax 70 energy-dispersive X-ray system. The analysis confirmed the expected stoichiometric Mo:Se ratio in the crystals. Device fabrication After mechanical exfoliation of MoSe 2 monolayers on SiO2 substrates, a JEOL JBX-6300FS EBL system was used to pattern contacts in a 300-nm bilayer PMMA resist. An e-beam evaporator was used to deposit 6/60 nm of Ti/Au followed by liftoff in hot acetone, cleaning in several IPA baths and drying under N2. Optical measurements All spectra were collected via a Princeton Instruments Acton 2500i grating spectrometer and an Andor Newton CCD (charge-coupled device), with samples in a helium-flow cryostat. For differential reflectance measurements, an Ocean Optics tungsten halogen white light source is reflected into a × 40 ultra-long working distance objective using a neutral density, achromatic beam splitter and then focused on the sample (~2 μm spot size). The reflected signal from the sample is collected by the objective and sent back through the beam splitter into the spectrometer. For PL measurements, a similar setup is used, except the neutral density beam splitter is replaced by a dichroic beam splitter appropriate for the laser wavelength and a laser line notch filter is inserted before the spectrometer. How to cite this article: Ross, J.S. et al. Electrical control of neutral and charged excitons in a monolayer semiconductor. Nat. Commun. 4:1474 doi: 10.1038/ncomms2498 (2013).